Longitudinal unzipping of 2D transition metal dichalcogenides Unzipping of the basal plane offers a valuable pathway to uniquely control the material chemistry of 2D structures. Nonetheless, reliable unzipping has been reported only for graphene and phosphorene thus far. The single elemental nature of those materials allows a straightforward understanding of the chemical reaction and property modulation involved with such geometric transformations. Here we report spontaneous linear ordered unzipping of bi-elemental 2D MX 2 transition metal chalcogenides as a general route to synthesize 1D nanoribbon structures. The strained metallic phase (1T′) of MX 2 undergoes highly specific longitudinal unzipping owing to the self-linearized oxygenation at chalcogenides. Stable dispersions of 1T′ MoS 2 nanoribbons with widths of 10–120 nm and lengths up to ~4 µm are produced in water. Edge abundant 1T′ MoS 2 nanoribbons reveal the hidden potential of idealized electrocatalysis for hydrogen evolution reactions at a competitive level with the precious Pt catalyst. Discovery of 2D atomic structures, including graphene, transition metallic dichalcogenides (TMDs), h -boron nitride, phospherene, and mxene, has unveiled new possibilities in materials science [1] . Unzipping of the basal plane is a general issue to uniquely control the material signatures of the 2D materials, as evidenced by the effective transformation of intrinsically metallic graphene into semiconductors, while unzipped into few-nanometer-wide graphene nanoribbons [2] . Chemical modification of abundant edge sites endowed from the geometric transformation as well as quantum state confinement provides generic opportunities towards the modulation of diverse physicochemical characteristics [3] . Despite the well-recognized advantages, however, reliable unzipping has been successful only for graphene and phosphorene thus far [2] , [4] , [5] . 2D TMDs (MX 2 ) are a unique family of bi-elemental compounds consisting of an atomic layer of transition metal (M = Mo/W) sandwiched between chalcogenide elements (X = S/Se/Te) [6] . Motivated from the prediction of ideally balanced binding characteristics for hydrogen, MX 2 is particularly promising for the electrocatalytic hydrogen evolution reaction (HER) without the use of precious metal catalysts [7] . Unfortunately, the abundant crystalline basal planes of MX 2 are catalytically inert and the HER activity principally originates from their unsaturated edges and defects. While the edge to surface ratio of 2D MX 2 is highly limited, a considerable amount of research efforts has been devoted to promote the active sites by the shape engineering of mesoporous defect-rich films and vertical nanoflakes, or heteroelement doping [8] , [9] , [10] , [11] , [12] . Alternatively, phase engineering by Li ion intercalation has been found to induce a transition from intrinsic semiconducting phase (trigonal prismatic, 2H) to strained metallic phase (distorted octahedral, 1T′), which can also enhance the HER activity accompanied by the increased electron mobility [13] . Nevertheless, in contrast with noble metal catalysts such as Pt nanoparticles, the electronic structure of atomically thin materials is strongly influenced by local electrochemical reactions. Molecular absorption during HER at MX 2 surface can dramatically reduce the conductivity of MX 2, which can subsequently slow down the reaction kinetics and reduce the overall current density [14] Thus, increasing the edge sites is essential for the optimal catalytic performance. Unfortunately, the intrinsic three-atom-thick nature and multi-elemental crystalline structures of 2D MX 2 poses challenges for the delicate shape engineering towards desired morphologies and structures [15] , [16] , [17] . Here, we introduce solution-phase unzipping of 2D MX 2 under aqueous condition as a general route to the production of edge-enhanced MX 2 nanoribbons (NRs). Synthesis and structural characterization of MX 2 nanoribbons Our unzipping is a two-step process consisting of the intercalation of bulk MX 2 with Li + ions (to obtain Li x MX 2 ) and subsequent ultrasonication in oxygenated water to form a stable suspension. Upon the ultrasonication, Li x MX 2 undergoes spontaneous exfoliation and longitudinal unzipping (more details are included in Methods section, Supplementary Fig. 1 ). The generality of this method has established with different 2D MX 2 samples, including MoS 2 , MoSe 2 , MoTe 2, and WSe 2 (Fig. 1 and Supplementary Figs. 2 – 4 ). Scanning electron microscopy (SEM) image presents the initiation of unzipping from the edge of bulk MoS 2 crystal (Fig. 1a, b ). A further propagation of the directional unzipping under ultrasonication creates fully unzipped MoS 2 nanoribbons (NRs) together with minor portions of residual nanosheets and layered flakes (Fig. 1c and Supplementary Fig. 5 ). Fig. 1: Unzipping of 2D MX 2 . SEM image of ( a ) unzipped MoS 2 after 5 min of ultrasonication displaying the initiation of unzipping from flake edge, ( b ) Magnified image for unzipped edge and ( c ) Fully unzipped MoS 2 displaying discrete MoS 2 NRs. Scale bars, ( a , c ) 0.5 and ( b ) 0.1 µm. d , e TEM image of isolated MoS 2 NRs. Scale bars, ( d ) 0.2 and ( e ) 0.1 µm ( f ) AFM image of MoS 2 NRs. Scale bar, 0.2 µm ( g ) Plot of NR length as a function of width measured by TEM of more than 400 MoS 2 NRs. h STEM image of MoS 2 NR. Inset is the lattice image with low beam exposure displaying 2a0xa0 symmetry and Mo terminated zigzag edge structure. Scale bars, 1.5 and 0.15 nm (inset). i Raman spectra of bulk MoS 2 , 1T’ MoS 2 sheets (MoS 2 S) and MoS 2 NRs. Full size image The NRs showed a great colloidal stability in aqueous media. It has been established from previous reports that chemically exfoliated MoS 2 dispersion in water has negatively charged MoS 2 layers with lithium cations and hydroxide anions (Li + +(MoS 2 ) x- +(1-x) OH − ) aq . The range of negative charge has been reported to be 0.15–0.25 per Mo atom, which ensures a great colloidal stability in aqueous media [18] , [19] . The discrete NRs showed an average length of 0.3 µm even though occasionally length up to 4 µm can also be seen. The width of NRs ranged from 10 to 120 nm (Fig. 1c–g , Supplementary Figs. 6 and 7 ). AFM measurement of MoS 2 NRs displayed thickness of 0.7–4.7 nm (Fig. 1f , Supplementary Fig. 5C ). Detailed investigation on the crystalline structures of MoS 2 NR verified 1T′ crystal lattice structures with Mo-zig zag edge structure (Fig. 1h and Supplementary Fig. 8 ). Notably, the 1T′ phase is unstable under electron beam exposure and thereby get relaxed to 1T and 2H structure under electron microscopy imaging (Supplementary Fig. 9 ) [20] . Raman spectrum of the MoS 2 NR displayed signature peaks for 1T′ phase at 156 (J 1 ), 228 (J 2 ) and 330 cm −1 (J 3 ) (Fig. 1i ) [21] , [22] . Interestingly, the peak for in-plane vibration mode at 383 cm −1 (E 1 2g ) is absent in the spectrum, indicating that out-of-plane vibration mode at 405.5 eV (A 1g ) is more excited, which indeed confirms the high density of edge sites [23] . Similar Raman spectra is observed for NRs prepared from other MX 2 samples (Supplementary Fig. 2 – 4 ). Additional evidence for the metallic nature of 1T′ MoS 2 NRs is obtained from four-probe hall-effect measurements. A thin film of NRs spin coated on Si/SiO 2 substrate showed resistivity of 1.68 × 10 −2 Ωcm (Supplementary Fig. 10A, B ). The resistivity of MoS 2 NRs is comparable to the 1T′ MoS 2 nanosheets prepared by hydrothermal synthesis (10 −1 Ωcm) and chemical exfoliation (10 1 –10 −2 Ωcm) but higher than those prepared by solid-state reaction (10 −3 Ωcm) and exfoliation with high-power forming-gas microwave plasma (8.6 × 10 −5 Ωcm) [24] , [25] , [26] , [27] , [28] . The relatively low electron mobility of MoS 2 NRs (2.7 × 10 −2 cm 2 V −1 s −1 ) suggests the presence of defects and vacancies as well as edge sites [6] , [29] . The linear I-V characteristics of MoS 2 NRs advocate ohmic behavior (Supplementary Fig. 10C ). The local electronic properties of a single MoS 2 NR is obtained by employing conductive AFM (c-AFM) measurement (Supplementary Fig. 10D ). The I-V measurement of an individual MoS 2 NR showed ohmic behavior (Supplementary Fig. 10E ). However, the current map image showed inconsistent current density on the NR with a scan rate of 0.7 Hz and applied voltage of 200 mV (Supplementary Fig. 10F ) indicating the instability of metallic 1T′ phase as evident from the STEM measurement (Supplementary Fig. 9 ). Thermal annealing can induce the phase transformation of MoS 2 NRs from metallic to semiconductor phase (Supplementary Fig. 11 ). The transformation progresses gradually upon a thermal annealing above 100 °C and almost completes at 400 °C. The 2H phase contribution has been increased to more than 93 ± 3% at 400 °C. Notably, a peak around 236 eV, representative of Mo 6+ 3d 5/2 , is absent in the XPS spectra indicating that the oxidation of Mo is minimal in the all samples (Supplementary Fig. 11A ). In addition, quenching of J 1 and J 2 and J 3 peaks is observed in the Raman spectra for the samples annealed above 100 °C (Supplementary Fig. 11B ). A 1g peak becomes increasingly prominent and in-plane vibration modes at 383 cm −1 (E 1 2g ) has been restored with annealing temperature. The characteristic MoS 2 excitonic A and B peaks (600–700 nm) and a sharp convoluted C&D excitonic peak (~420 nm) have gradually emerged as a function of annealing temperature in the absorption spectra, indication of phase change (Supplementary Fig. 11C ). An emergence of weak PL peak was detected around 656 nm in the photoluminance spectrum (Supplementary Fig. 11D ) of MoS 2 NRs annealed at 400 °C, which also supports the formation of semiconducting 2H phase [26] . Mechanism of MX 2 unzipping According to previous literature, oxygenation at the basal plane of MX 2 upon ambient condition has been reported not to be site-specific but randomized, and thereby generally leads to the etching in a disordered manner to yield random porous MX 2 structures [30] , [31] . Noteworthy that those previous works have focused on the 2H phase of MX 2 . As a control test, we repeated our experiment with the MoS 2 samples of pure 2H phase and mixed phase of 1T′ and 2H (Methods). The obtained exfoliated sheets are randomly etched and highly porous in nature in accordance with the previous works in contrast to longitudinal unzipped structures obtained from pure 1T′MoS 2 (Supplementary Fig. 12 ). Typical synthesis methods for 1T′MX 2 results in a mixture of 2H and 1T′ phase. However our optimized lithium intercalation method yield more than 90% 1T′ phase, which is found to be very critical for their basal plane unzipping (associated discussion is given in Supplementary notes and Supplementary Figs. 13 and 14 ) [7] , [32] . We have performed density functional theory (DFT) calculation and compared the oxygen binding energy at the surface of 1T′ and 2H phases (Fig. 2a, b and Supplementary Fig. 15A, B ) for a further understanding of the unzipping mechanism in different crystalline phases. Binding energy per oxygen atom (E BE ) is calculated by the equation; E BE = (E *O -(E * + nµ O ))/n, where E * and E *O denotes the energy of MX 2 with and without O atoms. µ O is the chemical potential of O atom evaluated as ½ µ O2 . 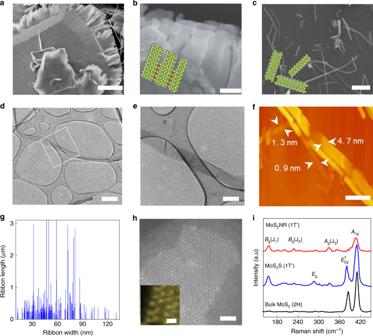Fig. 1: Unzipping of 2D MX2. SEM image of (a) unzipped MoS2after 5 min of ultrasonication displaying the initiation of unzipping from flake edge, (b) Magnified image for unzipped edge and (c) Fully unzipped MoS2displaying discrete MoS2NRs. Scale bars, (a,c) 0.5 and (b) 0.1 µm.d,eTEM image of isolated MoS2NRs. Scale bars, (d) 0.2 and (e) 0.1 µm (f) AFM image of MoS2NRs. Scale bar, 0.2 µm (g) Plot of NR length as a function of width measured by TEM of more than 400 MoS2NRs.hSTEM image of MoS2NR. Inset is the lattice image with low beam exposure displaying 2a0xa0 symmetry and Mo terminated zigzag edge structure. Scale bars, 1.5 and 0.15 nm (inset).iRaman spectra of bulk MoS2, 1T’ MoS2sheets (MoS2S) and MoS2NRs. Comparison of the E BE values at 1T′MX 2 surfaces for linear ordered vs. random arranged ones suggests a thermodynamic tendency towards a linearly ordered oxygenation (Table 1 ). By contrast, all 2H phases of MX 2 showed lower E BE values for random site oxygenation, in an agreement with the typical randomized etching. Investigation on such a preference for the longitudinal ordering in 1T′ phase by means of spin-resolved local density of states analysis showed the existence of two different types of X (S/Se/Te) sites (S1 and S2) with different electron densities (Fig. 2c and Supplementary Fig. 15C–E ). The S1 sites have a higher density of states at fermi level, and hence a stronger hybridization tendency can be anticipated between the p orbitals of X and oxygen compared to the S2 sites with a lower density of states. In the case of 2H phase, oxygen binding is randomized since such an asymmetry is absent (Fig. 2c ). Fig. 2: Oxygenation on the surface of MX 2 . a , b Difference in oxygen binding energies at 2H and 1T′ MoS 2 . While 2H phase prefers random binding of oxygen at surface, 1T′ phase prefers a linearized pattern. Insets show TEM images of randomly and linearly etched MoS 2 sheets. Scale bars, 100 nm. c The local density of states diagrams representing the similar (top) and different (bottom) density of states for S atoms in 2H and 1T′ phases. Full size image Table 1 Phase-dependent oxygenation. Full size table A strong alkaline pH is generally expected for the hydration of lithium intercalated MX 2 due to the generation of LiOH. Interestingly, the pH of the exfoliated solution drops drastically from alkaline (pH = 14.2) to acidic (pH = 3.4) upon the ultrasonication of Li x MoS 2 in oxygenated water (Fig. 3a ). We infer that the rapid decrease of pH upon ultrasonication should result from the dissolution of SO 2 released from the unzipping reaction (SO 2 + H 2 O ↔ H 2 SO 3 ). We evaluated the energies associated with the evolution of SO 2 /SeO 2 /TeO 2 species upon creating S/Se/Te vacancies in the basal plane of 1T′ phase to assess a simple thermodynamic aspect of this reaction route. All the formation energies were found to be negative (−3.59, −1.90, −1.20, and −1.60 eV for MoS 2, MoSe 2 , MoTe 2, and WSe 2 , respectively) indicative of the feasibility (Fig. 3b ). The longitudinal removal of XO 2 (SO 2 /SeO 2 /TeO 2 ) can be considered responsible for relatively low oxygen content in the resultant MX 2 NRs compared to etched 2H and mixed-phase MX 2 nanosheets (Fig. 3c and Supplementary Fig. 2 – 4D ). In addition, line faults are observed in SEM images of hydrated Li x MoS 2 (Supplementary Fig. 16 A–F). Interestingly, pH of the exfoliated solution did not show any significant drop upon ultrasonication of Li x WSe 2 in oxygenated water (Fig. 3a ). While scanning transmission electron microscopy (STEM) observation of partially unzipped MoS 2 identifies only MoS 2 (Supplementary Fig. 16D–F ), those of WSe 2 detects the by-product of Se (Fig. 3d–f ). This observation further confirms the evolution of XO 2 from the MX 2 surface since SeO 3 2− yielded from the dissolution of SeO 2 in water is known to undergo crystallization in basic conditions (SeO 3 2− +4e − +3H 2 O ↔ Se(↓)+6OH − ). Fig. 3: Mechanism for longitudinal unzipping. a Solution pH changes upon the ultrasonication of Li intercalated MoS 2 in oxygenated (Ox), deoxygenated (D.Ox), and deionized (D.I) water. Solution pH change upon hydration of Li intercalated WSe 2 in oxygenated water is also provided. b Schematic presentation of energetically favored removal of SO 2 from MoS 2 surface. c XPS analyses of Mo3d orbits of MoS 2 sheets of pure 2H phase and 2H:1 T′ combined phase and MoS 2 NRs prepared in oxygenated water. d – f HAADF and Elemental mapping (W, and Se) of partially unzipped WSe 2 layered sheet displaying Se as a byproduct and line defects on the basal plane. Scale bars, 0.2 µm. Full size image Notably, pH change is not prominent while Li x MoS 2 was ultrasonicated in deoxygenated or deionized water (Fig. 3a ). In addition, we did not observe any significant unzipping when 1T′ MoS 2 nanosheets (obtained by hydration of Li x MoS 2 in deoxygenated water) further ultrasonicated in oxygenated water. These results imply that the exothermic hydration of Li + supports the kinetics of XO 2 removal. A high concentration of dissolved oxygen can accelerate the removal of SO 2 creating chalcogenide vacancies during the hydration of Li x MoS 2 in water. Taken together, the underlying mechanism for the NR formation can be suggested as chemo-mechanical unzipping of MX 2 through the line faults created by chalcogenide vacancies under the sonochemical agitation of hot gas bubbles. Hydrogen evolution reaction performance of nanoribbons We have investigated the HER catalytic activity of MX 2 samples using a standard three-electrode electrochemical configuration in 0.5 M H 2 SO 4 electrolyte (Fig. 4 ). In order to investigate significance of unzipping, we compare HER activity of various MoS 2 samples. Figure 4a, b present the polarization curves and Tafel plots of MoS 2 samples, including 1D MoS 2 NRs unzipped from 1T′MoS 2 (MoS 2 NR), 2D 1T′MoS 2 sheets (1T′MoS 2 S), unexfoliated bulk 1T′MoS 2 (1T′MoS 2 B) and liquid phase exfoliated 2H MoS 2 porous sheets (2HMoS 2 PS). MoS 2 NR exhibits the highest HER performance even with a small loading (15 µg/cm 2 ), while attaining a current density ( j ) of 10 mA/cm 2 at very low potential (~79 mV versus RHE). 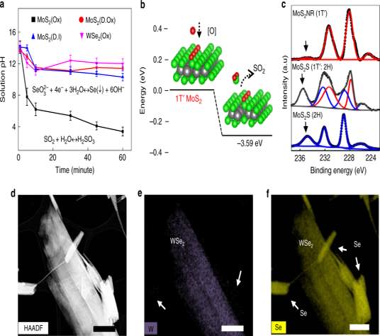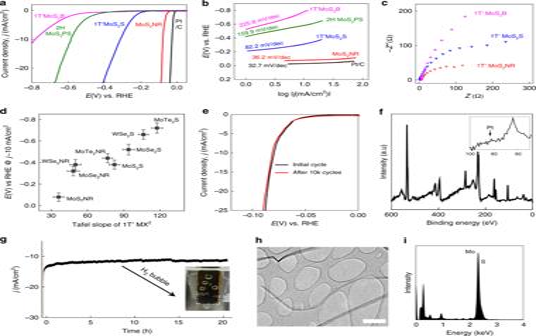Fig. 4: HER electrocatalytic activity of MX2NRs. aLinear sweep voltammograms and (b) corresponding Tafel plots for MoS2NR, 1T′ MoS2sheet (1 T′ MoS2S), 2H MoS2porous sheets (2H MoS2PS) and bulk 1T′ MoS2(1 T′ MoS2B). Pt/C is included as reference.cElectrochemical impedance spectroscopy data for MoS2NR, 1T′ MoS2S, and 1T′ MoS2B.dTafel slopes and required potentials to attain a current density of 10 mA/cm2for all unzipped 1T′ MX2NRs, compared to exfoliated 1T′ MX2S.ePolarization curves for MoS2NR before and after 10,000 CV scans.fXPS spectrum showing no Pt contamination during electrocatalytic cycling, inset is zoomed for 50–100 eV.gChronoamperometric response of MoS2NR at an applied potential of 80 mV vs. RHE displaying variation of current density up to 20 h. Inset shows photograph of H2bubbling on the electrode surface (h) TEM of MoS2NR catalyst after10000 cycles. Scale bar, 0.5 µm.iAssociated EDS spectrum. 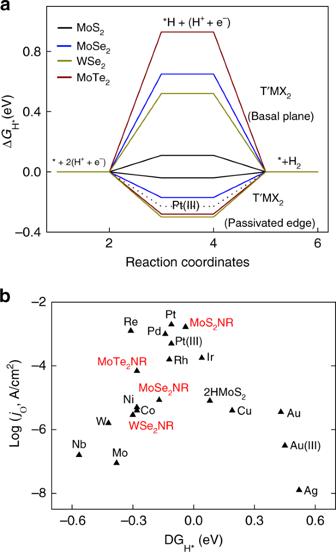Fig. 5: Theoretical investigation of HER of MX2NRs. aCalculated Gibbs free energy diagram for hydrogen binding at the basal plane and edge sites of 1T′ MX2systems at equilibrium potential (U = 0 V).bVolcano plot of the exchange current density vs. free energy for atomic hydrogen binding at MX2NRs and pure metal catalysts. Exchange current density of MX2NRs is normalized with the atomic site density of Pt for comparison. Fig. 3: Mechanism for longitudinal unzipping. aSolution pH changes upon the ultrasonication of Li intercalated MoS2in oxygenated (Ox), deoxygenated (D.Ox), and deionized (D.I) water. Solution pH change upon hydration of Li intercalated WSe2in oxygenated water is also provided.bSchematic presentation of energetically favored removal of SO2from MoS2surface.cXPS analyses of Mo3d orbits of MoS2sheets of pure 2H phase and 2H:1 T′ combined phase and MoS2NRs prepared in oxygenated water.d–fHAADF and Elemental mapping (W, and Se) of partially unzipped WSe2layered sheet displaying Se as a byproduct and line defects on the basal plane. Scale bars, 0.2 µm. Tafel slope and exchange current density is measured to be 36.2 mV/dec and 8.8 × 10 −6 A/cm 2 , respectively. 1T′MoS 2 S showed a better HER performance than 1T′MoS 2 B, verifying the significance of exfoliation of layered MX 2 for catalysis. Interestingly, 2HMoS 2 PS showed the lowest HER performance among all samples. Even with the high density of edge sites decorating random porous morphology, the low electrical conductivity of 2H phase is a bottleneck for the overall electrocatalytic activity. Noteworthy that MoS 2 NR showed lower resistance in the electrochemical impedance spectrum than 1T′ sheet due to the high charge transfer from the edge sites (Fig. 4c ). The annealed MoS 2 NRs showed a lower HER activity compared to 1T′MoS 2 NRs (Supplementary Fig. 17A ). This is in agreement with previous studies, which showed higher HER activity of 1T′ phase MoS 2 to corresponding 2H phase MoS 2 samples [33] , [34] . DFT studies have indicated that even though the free energy of hydrogen absorption of Mo-edge of 2H-MoS 2 is comparable to that of 1T′-MoS 2 , the kinetics of HER is restricted due to poor charge transfer in semiconducting 2H-MoS 2 leading to lower HER activity [35] . Fig. 4: HER electrocatalytic activity of MX 2 NRs. a Linear sweep voltammograms and ( b ) corresponding Tafel plots for MoS 2 NR, 1T′ MoS 2 sheet (1 T′ MoS 2 S), 2H MoS 2 porous sheets (2H MoS 2 PS) and bulk 1T′ MoS 2 (1 T′ MoS 2 B). Pt/C is included as reference. c Electrochemical impedance spectroscopy data for MoS 2 NR, 1T′ MoS 2 S, and 1T′ MoS 2 B. d Tafel slopes and required potentials to attain a current density of 10 mA/cm 2 for all unzipped 1T′ MX 2 NRs, compared to exfoliated 1T′ MX 2 S. e Polarization curves for MoS 2 NR before and after 10,000 CV scans. f XPS spectrum showing no Pt contamination during electrocatalytic cycling, inset is zoomed for 50–100 eV. g Chronoamperometric response of MoS 2 NR at an applied potential of 80 mV vs. RHE displaying variation of current density up to 20 h. Inset shows photograph of H 2 bubbling on the electrode surface ( h ) TEM of MoS 2 NR catalyst after10000 cycles. Scale bar, 0.5 µm. i Associated EDS spectrum. Full size image Indeed, the optimal integration of dense edge active sites with metallic 1T′ phase is unambiguously demonstrated by the excellent electrocatalytic HER kinetics for all MX 2 NRs (Fig. 4d , Supplementary Fig. 17B–E ). A comparison of electrochemical activities among the previously reported 2D MX 2 catalysts and our unzipped MX 2 is provided (Supplementary Table 1 ). Another critical feature for the viable HER catalyst is electrochemical stability. The HER polarization curve of MoS 2 NR displays no significant modification (ΔV = 3 mV @ 25 mA/cm 2 ) after a 10,000 cycling test, which verifies a long-term durability (Fig. 4e ). Notably, we did not observe any metal contamination even after 10,000 cycles (Fig. 4f ). MoS 2 NR shows a highly stable current density under continuous operation at 80 mV for 20 h (Fig. 4g ). Post catalysis characterization suggests that MoS 2 NRs can endure the long-term electrochemical stressing, as evidenced by the morphology or chemical state characterization (Fig. 4h, i ). The NRs displayed wrinkled morphology and slight aggregation, presumably due to the residual nafion contamination during electrode preparation, but well-maintained the 1T′ crystal structure (Supplementary Fig. 18 ). 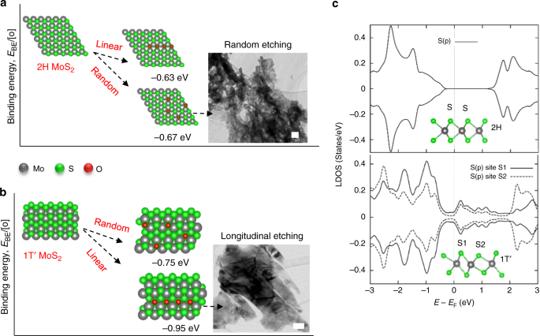We calculated the turnover frequency (TOF) to compare the intrinsic activity among various MX 2 NRs based on the assumption that only edge sites of MX 2 NRs are active for HER ( Supplementary notes ) [36] . After normalization with the typical active site density of Pt (1.5 × 10 15 sites/cm 2 ), we have calculated TOF of MoS 2 NRs to be 3.43 s −1 , higher than any previously reported molybdenum sulfide catalysts, including amorphous cluster (0.07 s −1 ), nanoparticles (0.02 s −1 ), vertical flakes (0.01 s −1 ), and sulfur vacant strained MoS x (0.31 s −1 ) [9] , [36] , [37] , [38] . Such a high TOF value of MoS 2 NR implies the existence of optimal catalytic sites even higher than Pt(III) surface (0.94 s −1 ) [36] . Fig. 2: Oxygenation on the surface of MX2. a,bDifference in oxygen binding energies at 2H and 1T′ MoS2. While 2H phase prefers random binding of oxygen at surface, 1T′ phase prefers a linearized pattern. Insets show TEM images of randomly and linearly etched MoS2sheets. Scale bars, 100 nm.cThe local density of states diagrams representing the similar (top) and different (bottom) density of states for S atoms in 2H and 1T′ phases. Other MX 2 NRs also showed favorable TOF values, including 0.017 s −1 for MoSe 2 , 0.142 s −1 for MoTe 2, 0.006 s −1 for WSe 2 (Supplementary Table 2 ). The high HER activity of MoS 2 NRs can be supported by the electrochemically active surface areas (ECSA), which were calculated from the double-layer capacitance (C dl ) obtained by cyclic voltammetry curves (Supplementary Fig. 19 ). Considering that ECSA is directly proportional to capacitance, MoS 2 NRs with a high C dl (10.1 mF/cm 2 ) attain the highest ESCA among the MX 2 NRs investigated in this study ( Supplementary notes and Supplementary Table 1 ). It is noteworthy that while edges play leading contribution, other factors, such as basal-plane activity should also have contributed to the overall activity of MX 2 NRs. Accordingly, we evaluated the HER activity of 1T′MX 2 using DFT by comparing the Gibbs free energy (ΔG H* ) for hydrogen adsorption at both basal plane and edge active sites. The calculation successfully predicts the highly active sites at the passivated edges of 1T′MX 2 compared to basal plane (Fig. 5a ). The ΔG H* close to zero at MoS 2 edge site (−0.04 eV) validates the highest HER activity of MoS 2 NR among all tested MX 2 NRs in this study. This is attributed to the relative electron deficiency of Mo sites arising from the stronger electronegativity of neighboring S atoms compared to other chalcogenides. For a quantitative comparison with the typical metal catalysts, a Volcano plot is prepared with the experimental exchange current density plotted against the DFT calculated ΔG H* [36] , [39] . While all MX 2 NRs well-follow the volcano trend, MoS 2 NR occupies the desirable position comparable to those of precious Pt group metals (Fig. 5b ). Fig. 5: Theoretical investigation of HER of MX 2 NRs. a Calculated Gibbs free energy diagram for hydrogen binding at the basal plane and edge sites of 1T′ MX 2 systems at equilibrium potential (U = 0 V). b Volcano plot of the exchange current density vs. free energy for atomic hydrogen binding at MX 2 NRs and pure metal catalysts. Exchange current density of MX 2 NRs is normalized with the atomic site density of Pt for comparison. Full size image We have demonstrated with the help of DFT studies a phase-dependent oxygenation pattern in 2D MX 2 . While 2H phase MX 2 undergoes oxygenation at random positions, the oxygenation in 1T′ MX 2 is linear ordered due to the presence of two types of chalcogenides with different electron densities. In contrast to typical chemisorption, chalcogen atoms are removed in the form of XO 2 (SO 2 , SeO 2 , and TeO 2 ) during the oxygenation process creating line faults under the exothermic hydration of Li x MX 2 in oxygenated water. Sonochemistry and agitation of ultra-hot gas bubbles involved in the sonication cause the chemo-mechanical unzipping of 1T′ MX 2, which initiates and propagates through these line faults. Abundant active edges decorating the 1T′ NRs serve for the well-balanced molecular binding sites for optimal HER catalyst. This effective geometric transformation exploiting delicate surface reactivity control highlights how to tailor the nanoscale morphology of polymorphs of low-dimensional multi-element structures. Thus, a broad spectrum of potential functionalities depending on diverse choices of chemical compositions can be extrapolated. Synthesis of lithium intercalated MX 2 (LixMX 2 ) Bulk MX 2 (MoS 2 , WSe 2 , and MoSe 2 ) flakes of 99.8% purity were purchased from Alfa Aesar. MoTe 2 crystals were purchased from Sigma Aldrich and ground to powder. All samples were first degassed by keeping under vacuum at 60 °C for 48 h. Degassed MX 2 (100 mg) was treated with different concentrations of n -butyl lithium ( n -BuLi) (stock concentration of 1.6 M, Sigma Aldrich) in hexane at a fixed dose of 10 mg/ml under different temperature from 20 to 120 °C. The treatment time was varied from ~6 to 100 h to synthesize Li x MX 2 . After a predetermined intercalation time, the suspension was filtered over Millipore membrane and washed several times with high purity hexane to separate the intercalated MX 2 from residual n -BuLi. The entire procedure was carried out in a glove box under extra pure N 2 atmosphere. Since lithium compounds react violently in the presence of humid air, dealing with a large amount of Lithium compounds requires cautious treatment. We have made several small batches (2 ml) inside the N 2 -filled glove box to acquire a sufficient amount of materials for this study. Synthesis of 2D MX 2 sheets (MX 2 S) To prepare MX 2 S sheets of pure 1T′ and 1T′:2H combination phase (associated discussion is in Supplementary file and supplementary Figs. 13 and 14 ), purified Li x MX 2 was exfoliated in deionized water by ultrasonication for 2 h. The solution was then slowly dropped into a hexane column (3000 ml) at a rate of 0.1 ml/minute to wash away any organic residues. The recovered solution from the hexane column is then centrifuged several times in high purity deionized water to remove the impurities and unexfoliated MX 2 . The aliquot was recovered to obtain exfoliated MX 2 sheets. To prepare unexfoliated bulk 1T′ MX 2 (1 T′ MX 2 B), purified Li x MX 2 was hydrated in deionized water without ultrasonication to prevent exfoliation. Pure 2H phase exfoliated MX 2 sheets (2HMX 2 S) were obtained by liquid phase exfoliation. In a typical procedure, bulk MX 2 (1 mg/ml) was ultrasonicated in a mixture of ethanol-water (1:1; v;v) for 1 h and centrifuged to recover the aliquot containing exfoliated 2HMX 2 sheets. The exfoliated MX 2 sheets in ethanol water mixture is solvent exchanged to oxygenated water by further centrifugation and redispersion procedures. This is then ultrasonicated for 2 h to investigate the oxygenation (2H MX 2 PS). Oxygenated water was prepared by purging O 2 gas of 99.9% purity directly into 200 ml of deionized water in a closed glass vessel for 1 h. In order to prepare the deoxygenated water, 200 ml of deionized water was placed in a stoppered Buchner flask attached to a vacuum pump. The water was heated to 60 °C with magnetic stirring for 1 h under vacuum to get rid of all the dissolved oxygen in the deionized water. Unzipping of MX 2 After intercalation reaction with optimized conditions to achieve pure 1T′ phase, the recovered Li x MX 2 was transferred to a vessel containing oxygenated water. The suspension was ultrasonicated and dropped into a hexane column (3000 ml) at a rate of 0.1 ml/min to wash away n -BuLi residue. Afterwards, the recovered suspension of MX 2 in water from the bottom of the hexane column was further diluted in oxygenated water (300 ml) and ultrasonicated for 2 h. The suspension was aged sufficiently before centrifugal separation (20,000 rpm for 2 h) to recover the unzipped MX 2. The obtained MX 2 NRs was redispersed in ethanol or water and centrifuged several times from 8000 to 3000 rpm, each time discarding the sediments to remove the unexfoliated and partially unzipped MX 2 . Noteworthy that only ~2.0 ± 1.4% of the starting material was retained in the supernatant. The majority of raw material was etched away and/or remained as bulk layered structures that could be removed by centrifugation. We found that a prolonged sonication does not lead to a higher yield of NRs. The sonication time was carefully controlled to ~2 h for the optimal yield of NRs. Note that, the experimental conditions described here such as initial Li ion concentration, temperature, reaction time, sonication time, and purification steps may change depending on the crystal quality and flake size of precursor source. The aliquot recovered after centrifugation was drop-casted on Cu-carbon grids for TEM and STEM measurements and Si/SiO 2 substrate for XPS and Raman measurements. For HER electrode preparation, the aliquot was vacuum dried under N 2 at 40 °C. Characterization of MX 2 NRs TEM, HRTEM, and EDS were performed with field emission TEM of 200 kV (Talos F200x, Tecnai F20, FEI). HAADF-STEM characterization was carried out with a double-aberration corrected HRTEM (Titan G2 60–300, FEI) at 80 and 200 kV accelerating voltage. SEM imaging was obtained with ultra-high resolution field emission scanning electron microscope (Hitachi, SU8230). Optical microscope (Olympus, Japan) was used for the optical imaging. Raman and XPS spectra were recorded with ARAMIS (Horiba Jobin Yvon) and k-alpha (Thermo VG Scientific), respectively. Hall Effect measurements and I-V curves were obtained using Ecopia Hall Effect measurement system (HMS-3000) equipped with spring clipboard sample mounting boards (SPCB) containing four gold plated pins. NRs were spin coated on the Si/SiO 2 substrates and directly mounted on the SPCB. The distance among pins was fixed as 5 mm. Silver paste was used to make a good ohmic contact between the pin and the sample. Conductive AFM (MFP-3D, Asylum Research) measurement was carried out with Cr/Pt-coated cantilevers (ConEG, Budget Sensors) and Cr/Au-coated Si substrate. A three-electrode electrochemical cell was used for the electrochemical measurements with a Bio-Logic, SP-200 potentiostat. MX 2 deposited glassy carbon electrode acted as the working electrode with a Pt wire as the counter electrode and a saturated calomel electrode as a reference electrode. Known weights of MX 2 samples (15 µg) dispersed in ethanol were directly deposited onto the working electrode using a micropipette and dried at 60 °C under N 2 flow. 10 µl of 5% Nafion was deposited as a protective layer on the surface of sample placed on glassy carbon electrode. Any incidence of Pt contamination was ruled out by repeating the same experiments with carbon counter electrode. Calibration of the reference electrode to reversible hydrogen electrode potential (RHE) was conducted in 0.5 M H 2 SO 4 electrolyte with Pt wire as both counter and working electrode and found to be E RHE = E SCE + 0.252 V. The electrolyte was constantly stirred by a magnetic stirrer during an electrochemical test to facilitate mass transport and prevent the accumulation of bubbles on the surface of electrode. Details of measurements and calculation of Tafel slope, ESCA, and TOF values are provided in the supplementary information. Computational details Spin-polarized density functional theory (DFT) computations were performed using the Vienna Ab-initio Simulation Package (VASP) with the projector-augmented-wave (PAW) method to account for core-valence interactions. Details of calculations are provided in the supplementary information. STEM image simulations were obtained using an open-source software QSTEM [40] .